Multistability and switching in a superconducting metamaterial The field of metamaterial research revolves around the idea of creating artificial media that interact with light in a way unknown from naturally occurring materials. This is commonly achieved using sub-wavelength lattices of electronic or plasmonic structures, so-called meta-atoms. One of the ultimate goals for these tailored media is the ability to control their properties in situ . Here we show that superconducting quantum interference devices can be used as fast, switchable meta-atoms. We find that their intrinsic nonlinearity leads to simultaneously stable dynamic states, each of which is associated with a different value and sign of the magnetic susceptibility in the microwave domain. Moreover, we demonstrate that it is possible to switch between these states by applying nanosecond-long pulses in addition to the microwave-probe signal. Apart from potential applications for this all-optical metamaterial switch, the results suggest that multistability can also be utilized in other types of nonlinear meta-atoms. In recent years, the idea of using superconducting quantum interference devices (SQUIDs) and their quantum analogues (qubits) as meta-atoms in superconducting microwave metamaterials has become increasingly appealing as the attention of the community shifts towards tunability and parametric effects [1] , [2] , [3] , [4] . In the quantum limit, efforts to build many-qubit systems blur the border between circuit quantum electrodynamics and metamaterials [5] , [6] , [7] , [8] while even the classical case holds a multitude of interesting and yet unexplored possibilities. Implementations of these structures, for instance in the form of parametric amplifiers [9] , have already attracted a great deal of attention and continue to do so as the field of superconducting metamaterials evolves. In the present work, we are focusing on an effect found in single-junction (radio frequency (rf-))SQUIDs. To some extent, they are similar to split-ring resonators, one of the most common meta-atom designs, as they consist of a (superconducting) loop interrupted by a Josephson tunnelling barrier instead of a capacitor. Although superconductivity and the Josephson effect are quantum phenomena, the way the SQUIDs are built and operated allows us to describe them using classical dynamic equations, as one would model other resonant meta-atoms. Unlike other resonant meta-atoms, however, they exhibit a unique dependence of their resonance frequency on a constant, external magnetic field. It stems from the nonlinear nature of the Josephson junction. This effect has been widely discussed [10] , [11] , [12] and demonstrated in different waveguide geometries [13] , [14] , [15] Although this truly remarkable feature is a direct effect of the Josephson nonlinearity, the SQUIDs in the cited experiments were mostly operated at excitation powers low enough to treat the junction as a quasi-linear inductive element. With increasing power, this simple model fails as the nonlinearity starts to influence the resonant behaviour. So far, this regime has not been explored in great detail experimentally. The essence of this work is the dynamic multistability which occurs in non-hysteretic rf-SQUIDs at intermediate power levels where the linear treatment starts to fail. This has already been observed in single junctions [16] and investigated numerically for rf-SQUID meta-atoms [17] . It should be noted that here, we deal with a purely dynamic phenomenon that is not related to the multistability known from hysteretic SQUIDs [18] , [19] . For a certain choice of parameters, the dynamic multistability manifests itself as a small number of simultaneously stable states, each of which corresponds to a different value of the SQUIDs’ magnetic-flux susceptibility χ ϕ at the driving frequency. More importantly, a closer analysis reveals that in many cases coexisting stable states have small-positive as well as large-positive and large-negative values of the real part of χ ϕ . This means that, depending on the current state of the meta-atom, it can either be magnetically almost transparent, strongly enhance the local-magnetic field by oscillating in phase with the drive, or even counteract the same by oscillating out of phase. This is a highly desirable feature for a meta-atom provided one can reliably switch it from one to another state in situ . Similar to the quantum switch [20] and unlike most other switchable meta-atoms, the process of switching in this approach is not associated with a change of the static mechanical [21] or electronic [22] properties. Here, we demonstrate the switchability of the SQUIDs experimentally and provide an analytical model describing the observed behaviour. Finally, we show how a chain of these meta-atoms can be implemented as a metamaterial device. Switching by microwave pulses The most prominent feature associated with the effect described below is that it is possible to switch between the states reproducibly by applying a short-microwave pulse to the metamaterial. To verify this experimentally, we used a coplanar waveguide (CPW) loaded with a one-dimensional (1D) metamaterial consisting of 54 rf-SQUIDs. A row of 27 SQUIDs is located in each of the two gaps of the CPW. The coupling between the waveguide and the SQUIDs is designed to be primarily magnetic, which is why a change in the magnetic susceptibility seen by the waveguide can be measured as a change in its scattering characteristics. 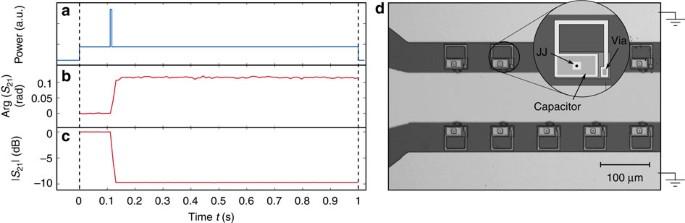Figure 1: Switching of a 54 SQUID array. (a) Sketch of the pulse sequence used to switch the 1D metamaterial. The actual measurement, indicated by two vertical dashed lines, takes place after initializing the system in a small amplitude state. (b) Transmission phase and (c) magnitude measurement of the SQUID-loaded waveguide recorded as a function of time. The steepness of the jump is limited by measurement bandwidth. The base-line has been subtracted for both curves. The pulse switches the system into another stable, dynamic state which is visible as change in transmission. (d) Microscope image of a section of the loaded CPW and a close up sketch of a single SQUID. The arrow in the round inset labelled JJ marks the position of the Josephson junction. Figure 1 shows an exemplary transmission measurement recorded in such an experiment. Initially, the system is in a state with a susceptibility close to zero which results in little scattering and thus a large transmission through the loaded CPW. By applying the microwave pulse, the system is driven into a state with | χ ϕ | ≫ 1 which results in both enhanced reflection and absorption of the probe signal. Together, this causes the amount of transmitted power to drop by one order of magnitude (10 dB) for this sample. The system remains stable in the new state until it is reset. Figure 1: Switching of a 54 SQUID array. ( a ) Sketch of the pulse sequence used to switch the 1D metamaterial. The actual measurement, indicated by two vertical dashed lines, takes place after initializing the system in a small amplitude state. ( b ) Transmission phase and ( c ) magnitude measurement of the SQUID-loaded waveguide recorded as a function of time. The steepness of the jump is limited by measurement bandwidth. The base-line has been subtracted for both curves. The pulse switches the system into another stable, dynamic state which is visible as change in transmission. ( d ) Microscope image of a section of the loaded CPW and a close up sketch of a single SQUID. The arrow in the round inset labelled JJ marks the position of the Josephson junction. Full size image One noteworthy difference when comparing this system with other switchable metamaterials is that here, the switching process is rather fast because it only relies on the intrinsic properties of the nonlinear resonator. Thus the time required to switch is proportional to the decay time τ d =2 RC which is of the order of a few nanoseconds for our samples. Here, R and C are the intrinsic resistance and capacitance of the SQUID meta-atom, respectively. Experimentally we were able to verify that the switching takes place for pulses as short as 2 ns. Analytical modelling To better understand and predict the existence of the multiple stable, dynamic states, we developed an analytical model that is able to quantitatively reproduce most of the experimental observations. We start from the basic differential equation that defines the evolution of the total gauge-invariant phase difference φ over the Josephson junction of the SQUID when driven externally by φ ext . where , , , , I c is the maximum supercurrent that can be carried by the Josephson junction, C is the capacitance shunting the junction, L is the inductance of the loop, and R is the damping. Assuming a harmonic drive φ ext = φ ea cos ω t , we can make an ansatz for the solution of the equation of motion: φ = x cos( ωt )− y sin( ωt ). This corresponds to all harmonic solutions that have an amplitude and a phase δ =arctan( y / x ) with respect to the drive. The magnetic-flux susceptibility can then be defined as the time average of the ratio between the flux in the loop and the driving flux which can be expressed as χ φ =〈 φ / φ ext 〉 t −1. It should be noted at this point, that it is not obvious that this approach will describe the dynamics of the system sufficiently well, because it does not contain contributions from higher harmonics. A detailed treatment of why this approximation is applicable in our case is provided in the methods section. Using the mentioned ansatz, one can write down the equations of motion in the rotating-wave approximation (RWA) together with the stability condition: Here, g is the potential in the rotating frame [23] : where J 0 is the zeroth order Bessel function of the first kind. These equations yield both stable and unstable solutions which can be distinguished from each other through a stability analysis. 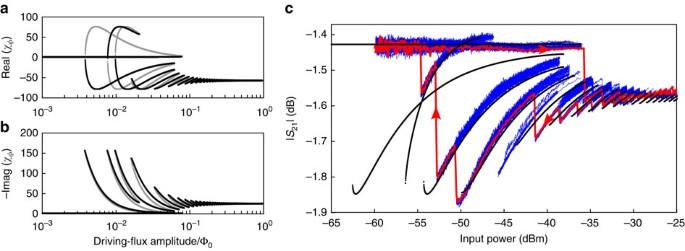Figure 2: Multistability of a single SQUID. (a) Real and (b) imaginary part of the magnetic-flux susceptibility of a single SQUID meta-atom calculated from equations (2)–(4), , . Stable solutions are shown in black, while unstable solutions are in grey. (c) Calculated (black) and measured (blue and red) transmission through the sample arrangement containing only a single SQUID. The red data show a hysteresis loop from low to high power and back. The red arrows indicate the direction of the sweep. The blue data are a collection of different power sweeps of varying length and initial conditions. The overall transmission of less than −1.4 dB is caused by the experimental setup and calibration and not related to the performance of the meta-atom. Figure 2a,b shows the real and imaginary part of the calculated magnetic-flux susceptibility for a fixed frequency as a function of the amplitude of the drive. For a certain range of driving power, multiple stable (black) and unstable (grey) solutions coexist. Moreover, the simultaneously stable states can have a small-positive as well as a large-negative and a large-positive values of the real part of χ ϕ . These results can then be used in a transmission-line approach to calculate the transmitted power through the sample as seen in Fig. 2c (black line). Qualitatively, this effect exists for a wide range of frequencies and magnetic field values, however with varying magnitude. Here, we focus on a region slightly above the LC-resonance frequency where the effect is most pronounced. Figure 2: Multistability of a single SQUID. ( a ) Real and ( b ) imaginary part of the magnetic-flux susceptibility of a single SQUID meta-atom calculated from equations (2)–(4), , . Stable solutions are shown in black, while unstable solutions are in grey. ( c ) Calculated (black) and measured (blue and red) transmission through the sample arrangement containing only a single SQUID. The red data show a hysteresis loop from low to high power and back. The red arrows indicate the direction of the sweep. The blue data are a collection of different power sweeps of varying length and initial conditions. The overall transmission of less than −1.4 dB is caused by the experimental setup and calibration and not related to the performance of the meta-atom. Full size image The fact that multistability only occurs in a limited range of driving power [24] can be understood from the particular form of the Josephson nonlinearity sin φ in equation (1). For very small-driving amplitudes, this term can be linearized around a static phase value φ const which is in turn related to the direct current (DC) magnetic flux seen by the SQUID loop. Therefore, the SQUID is usually treated as a DC-flux tunable, quasi-linear resonator in this driving regime. For very large-driving amplitudes the nonlinear term in equation (1) is strongly suppressed. As a result, the system can be described as a DC-flux independent LC circuit resonating at f LC in this regime. Consequently, the only case in which the nonlinearity contributes to the dynamic behaviour of the system is in the intermediate range of driving amplitudes. Our analysis also shows that both the number of observable states and their amplitudes strongly depend on the difference between driving frequency and f LC . Multistability in a single SQUID To test the analytical model and verify the existence of the dynamic states, we demonstrate two ways of measuring them: by sweeping power up and down thus going through a hysteresis loop and by exciting the system using microwave pulses. We first demonstrate the hysteresis (red curve in Fig. 2c ) for a single SQUID meta-atom to obtain results that can be compared directly with the single SQUID analytic solution. At a low initial-power level, the systems starts out in a transparent state (small absolute value of χ ϕ ) resulting in a large value of the transmission | S 21 | through the SQUID-loaded CPW. When increasing the power, it remains in this state until it is no longer stable (≈−37 dBm in this case). The system then settles in one of the excited states (large-absolute value of χ ϕ ), which results in a drop in the transmitted power. Following a series of small jumps, the system eventually reaches a stable level. Upon sweeping the power back, the observed transmission takes a different path by following several of the highly excited states until they become unstable then jumping to the closest stable one. Although being consistent with the model, this method only reveals a small fraction of the predicted-stable states. For a more complete picture one can prepare the system in each of the states using the hysteresis and then follow each path in both directions until it becomes unstable. The resulting curves are shown as blue lines in Fig. 2c . One noteworthy aspect in this figure is that all but one of the highly excited states correspond to solutions with a negative-real part of χ ϕ as seen in Fig. 2a . The only solution with a large-positive real part of χ ϕ in Fig. 2a corresponds to the line that crosses the base-line at about −50 dBm driving power in Fig. 2c . Although the data agree with the theoretical prediction to a quantitative level in many aspects, there is still a slight discrepancy between the two. The most noticeable difference is that even by varying the initial conditions for each sweep, we are not able to prepare the system in all states predicted by the model. Multistability in SQUID arrays As mentioned above, this approach can be extended from a single meta-atom to a metamaterial. In this case, however, even without any disorder, the multistability will not have such a clear signature in transmission measurements any more. This is owing to the fact that the probe signal gets absorbed and reflected as it passes through the 1D metamaterial so that every meta-atom sees a different effective input power. In case of the 1D 54 SQUID array, one can still observe the characteristic hysteresis loop (blue curve in Fig. 3 ) albeit without the distinct response of the different states. Figure 1 shows that in this case, it is possible to decrease the transmission by up to 10 dB by applying a short-microwave pulse. With the knowledge of the theory and the hysteresis curve, the pulse sequence shown in Fig. 1a becomes clear: the first part is necessary to reset the system to the transparent state. The intermediate power level (usually just referred to as input or driving power) moves the system to the multi-stable power region, while keeping it in the transparent branch. Finally, the pulse excites the system into a different branch of the hysteresis. The decrease in transmission thus depends on the input-power level and is subject to a statistical spread. A more detailed overview of the switching as a function of the input power is given in Fig. 3 . The black points show the mean magnitude of the difference in | S 21 | before and after applying the microwave pulse and its standard deviation. Each of the points contain information from 150 measurements using the sequence outlined in Fig. 1 . Apart from the driving-power level, the switching also depends on duration and amplitude of the pulse, all of which influence the number of switched SQUIDs in the array and thus the resulting change in transmission. Ideally, the magnitude of the switching should follow the difference between the up- and down-sweep branches of the hysteresis. For the combination of parameters chosen in Fig. 3 (pulse duration: 200 ns, pulse power at the sample: −38 dBm), however, the switching only works reliably in part of the input-power range (between −58 dBm and −52 dBm). 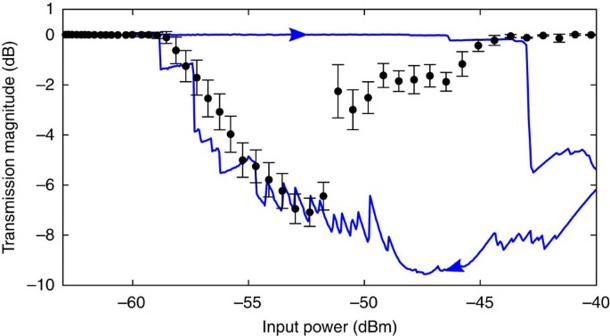Figure 3: SQUID-array results. Hysteresis curve for a CPW loaded with 54 SQUIDs (blue line) normalized to the value at −65 dBm. The black dots show the mean magnitude and standard deviation (150 samples) of the difference in |S21| before and after applying a microwave pulse. Up to about −58 dBm this quantity is well-described by the difference between the lower and upper branch of the hysteresis. Above that threshold, the switching magnitude drops to a lower value. Figure 3: SQUID-array results. Hysteresis curve for a CPW loaded with 54 SQUIDs (blue line) normalized to the value at −65 dBm. The black dots show the mean magnitude and standard deviation (150 samples) of the difference in | S 21 | before and after applying a microwave pulse. Up to about −58 dBm this quantity is well-described by the difference between the lower and upper branch of the hysteresis. Above that threshold, the switching magnitude drops to a lower value. Full size image The presented results demonstrate the general possibility of creating an on-chip metamaterial switch from switchable meta-atoms. As such, its performance (on/off ratio of about 10:1 and limited dynamic range) can be questioned. With the current design of identical SQUIDs there is indeed a limit to those quantities. The performance of the device is related to the hysteresis curve of the single SQUID. This relation can qualitatively be summarized as follows: when all SQUIDs are in the transparent state, they all see the same amount of driving power since the scattering at every meta-atom is small. However, as soon as some of the SQUIDs are switched to a different state, they absorb and reflect part of the microwave drive, so the ones located behind them (in propagation direction) feel a weaker drive. In a long chain of SQUIDs a situation will eventually be reached in which the elements further back in the chain are biased outside of their hysteresis range. Thus the limit of the switching magnitude of the array is given by the width of the hysteresis curve of a single SQUID as seen in Fig. 2 . Some options to improve upon the basic design include optimizing the individual SQUIDs (in terms of width and onset of the hysteresis) and making them non-identical. Despite the aforementioned restrictions we believe that this approach presents a viable alternative to other switching techniques for the following reasons: first, the device can be switched by comparatively short, low-power pulses and remains stable with a high fidelity. Second, it can easily be integrated with other technology based on Josephson junctions such as qubits or Josephson parametric amplifiers. Third, the concept can directly be extended into two or three dimensions by arranging SQUIDs accordingly thus making a pulse-switchable surface or 3D body. We would also like to point out that, although the nature of the Josephson junction is responsible for this particular shape of the multistability, the way it is implemented here is of a more general nature. Switching the oscillatory state of a meta-atom by means of pulses can be extended to other types of nonlinearites and different technologies that do not require superconductivity [25] . In conclusion, we have implemented and demonstrated a 1D metamaterial consisting of switchable meta-atoms. By operating non-hysteretic, single-junction SQUIDs in an intermediate power range, we showed that they can be switched between different dynamic states corresponding to different values of their magnetic susceptibility. For individual meta-atoms, we were able to map these states directly in a transmission experiment. We developed an analytical model based on the rotating-wave approximation which shows excellent agreement with the measured data. Using an array containing 54 SQUID meta-atoms, we showed that one can switch the transmission through this 1D metamaterial by applying a nanosecond-long microwave pulse. Unlike in other switchable meta-atom implementations, we employ an intrinsic nonlinearity which makes these SQUIDs very fast-switching meta-atoms. The samples The SQUIDs are thin-film Nb structures with a Nb-AlO x -Nb tunnel barrier. They are ∼ 45 × 49 μm 2 in size with a 2 μm 2 junction area which is shunted by a large Nb 2 O 5 capacitor. They are positioned in the gaps of a CPW on a 4 × 4 mm Si chip. The values used to model the SQUIDs are ω p =5.276·10 10 s −1 , ω c =5.438·10 12 s −1 , β L =0.45. Experimental setup All measurements were performed in liquid 4 He at a temperature of 4.2 K using cryogenic amplification. The sweeps were recorded with a vector network analyzer. Pulses were generated using a microwave mixer and a pulse generator. Data calibration The measurements were thru-calibrated at the connector closest to the sample. Additional scatterers that could not be calibrated out this way (that is, bond-connections) were accounted for whenever theory and experiment were compared. Validity of the RWA In general, the solution for the phase φ is of the form, In equation (1), we only keep the resonant components y 1 = y and x 1 = x according to the rotating-wave approximation. Since the anharmonicity is relatively large, we also want to explicitly control the validity of this approximation. If we go beyond the rotating-wave approximation not only the first mode, oscillating with frequency ω, will be excited but also higher modes. The closer the higher the modes are to the first mode, the stronger they should be excited. Therefore, we keep the second and third mode oscillating at 2 ω and 3 ω , respectively. In this case, the quasi-energy Hamiltonian takes the form where y 0 is the conjugate variable of x 0 , J n the nth order Bessel functions of the first kind and we assumed that x n and y n remain small for n =2, 3. The resulting equations of motion for n ≥1, are given by And for n =0 we get Equation (9) has a stationary state ( ) for x 0 =0 independent of x 1 and y 1 . In this case we only have to consider the coupling between the resonant mode and x 3 , y 3 because the first mode will not couple to the second mode. Using the lowest order of perturbation theory we calculate the solution for x 1 and y 1 as discussed above and find an order of magnitude estimate from the stationary equation of motion: Solving this, we get for the amplitude of the oscillations of the third mode On resonance we have , thus we can simplify the expression to The ratio between the amplitude of the third harmonic to the amplitude at the driving frequency A 3 / A 1 is a useful figure to quantify the validity of the RWA. We can find an upper limit for this quantity since the Bessel function divided by its argument can be estimated by | J 3 ( A 1 )|/ A 1 <1/9 and β L <1/2. Thus A 3 / A 1 <1/144 which means that the rotating-wave approximation is well justified. The frequency range of interest for the experiment at hand is determined by the low-power tuning range of the resonance frequency which is bounded by from above and from below. In this frequency range the ratio is A 3 / A 1 <1/63, which is still well within the regime of the rotating wave approximation. How to cite this article: Jung, P. et al. Multistability and switching in a superconducting metamaterial. Nat. Commun. 5:3730 doi: 10.1038/ncomms4730 (2014).